Reply to: “Inconsistent prediction capability of ImmuneCells.Sig across different RNA-seq datasets” 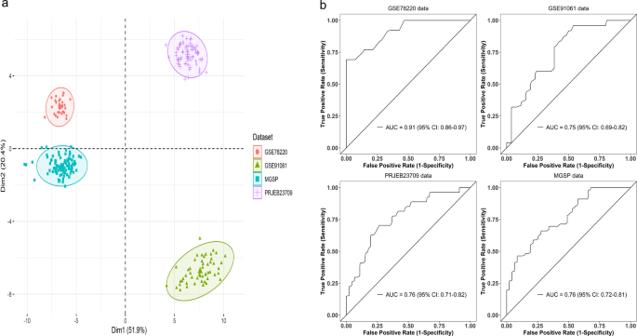Fig. 1: Divergence between different data sets and the fivefold cross-validation of ImmuneCells.Sig across the data sets. aFirst two principal components of all individuals from data sets GSE78220, GSE91061, PRJEB23709, and MGSP.bThe fivefold cross-validation showed that the ImmuneCells.Sig still had good predictive values across the independent data sets. The plots of the results of the mean testing AUC values for each of the four data sets were shown, i.e., for GSE78220, GSE91061, PRJEB23709, and MGSP data sets. 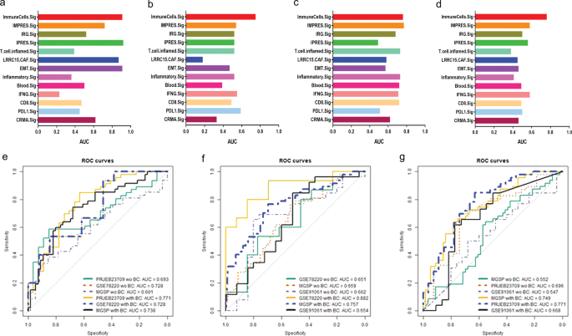Fig. 2: Comparison of the performance of ImmuneCells.Sig with other ICT (immune checkpoint therapy) response signatures and independent validation of ImmuneCells.Sig without or with batch effect correction. The multiple bar plots of the fivefold cross-validation calculated mean testing AUC (Area Under The Curve) values of the whole 13 ICT signatures are shown inaFor the GSE78220 data set.bFor the GSE91061 data set.cFor the PRJEB23709 data set.dFor the MGSP data set.eTesting the predictivity of the ImmuneCells.Sig trained in the GSE91061 data set in the other three independent data sets—PRJEB23709, GSE78220, and MGSP without or with batch effect correction.fTesting the predictivity of the ImmuneCells.Sig trained in the PRJEB23709 data set in the other three independent data sets—GSE78220, MGSP, and GSE91061 without or with batch effect correction.gTesting the predictivity of the ImmuneCells.Sig trained in the GSE78220 data set in the other three independent data sets—MGSP, PRJEB23709, and GSE91061 without or with batch effect correction. Principal component analysis and batch effect correction The four bulk RNA-seq data sets (GSE78220, GSE91061, PRJEB2370922, and MGSP), our self-developed gene expression signature—ImmuneCells.Sig and the twelve other published gene expression signatures for comparison in our original publication [1] were also used in this study. Principal Component Analysis (PCA) was conducted using the factoextra R package v1.0.7. To correct the batch effect, we utilized the removeBatchEffect function in the limma package v3.44.3 implemented in the R software package v3.6.3. Data analysis For validation study of the accuracy of the gene expression signature—ImmuneCells.Sig in predicting ICT outcome, we reanalyzed the data using the regularized logistic regression methods according to the previous studies [14] , [15] . The custom codes for applying the regularized logistic regression methods to our own data were developed based on the modification of the original codes kindly provided by Dr. Zhi-Ping Liu from a previous study [14] . Reporting summary Further information on research design is available in the Nature Research Reporting Summary linked to this article.